Approaching the limits of transparency and conductivity in graphitic materials through lithium intercalation Various band structure engineering methods have been studied to improve the performance of graphitic transparent conductors; however, none has demonstrated an increase of optical transmittance in the visible range. Here we measure in situ optical transmittance spectra and electrical transport properties of ultrathin graphite (3–60 graphene layers) simultaneously during electrochemical lithiation/delithiation. On intercalation, we observe an increase of both optical transmittance (up to twofold) and electrical conductivity (up to two orders of magnitude), strikingly different from other materials. Transmission as high as 91.7% with a sheet resistance of 3.0 Ω per square is achieved for 19-layer LiC 6 , which corresponds to a figure of merit σ dc / σ opt =1,400, significantly higher than any other continuous transparent electrodes. The unconventional modification of ultrathin graphite optoelectronic properties is explained by the suppression of interband optical transitions and a small intraband Drude conductivity near the interband edge. Our techniques enable investigation of other aspects of intercalation in nanostructures. Two-dimensional (2D) graphene has attracted much interest in fundamental research and technological development due to its extraordinary electrical, mechanical, thermal and optical properties [1] , [2] , [3] , [4] , [5] , [6] . Recently, graphitic films (from monolayer graphene to ultrathin graphite) have been explored as candidates for flexible transparent electrodes for electronics and optoelectronics [7] , [8] . An excellent performance of 30 Ω per sq at 90% transmittance has been achieved using doped four-layer chemical-vapour deposition (CVD) graphene [9] . Bulk materials with 2D-layered structures such as graphite have also been studied and used extensively for electrochemical energy storage based on intercalation [10] , [11] , [12] . Fundamental studies on intercalation in graphite have been extensively carried out [13] , and nanostructured 2D materials have recently gained much interest [14] . Reports on the intercalation of various species such as FeCl 3 (refs 15 , 16 ), Br [17] and Ca [18] in few-layer graphene (FLG) have offered a new route to designing and synthesizing graphene-based materials with novel conductive, magnetic or superconductive properties. It has long been known that the optical transmission of graphite increases on metallization by intercalation with, for example, caesium [19] . This unusual property results from the unique band structure of the graphene layer; intercalation heavily dopes ultrathin graphite, shifting the Fermi level upward more than any other band engineering method [15] , [19] , [20] , [21] , [22] , [23] , [24] , suppressing interband optical transitions due to Pauli blocking thus increasing transmittance of light in the visible range. The increase in optical transmittance is expected to be accompanied by an increase in conductivity since the carrier concentration increases on intercalation, an ideal situation for conductive transparent films. All studies to date of doped graphene films as transparent electrodes, however, do not report increased transmission in the visible range. It also has been assumed by some researchers that the transmission of ultrathin graphite can never exceed that of undoped graphene of similar layer numbers [25] . Moreover, no studies of electrical conductivity and optical transmission have been carried out for lithium-intercalated ultrathin graphite. Here, we use in situ electronic and optical measurements to understand the electrochemical intercalation process and simultaneously measure the electrical conductivity and optical transmission of exfoliated ultrathin graphite crystallites ranging from 3–60 graphene layers in thickness. On intercalation, we observe a large improvement in the optical transmittance, and at the same time a dramatic increase of sheet conductivity. The Dirac electronic band structure allows for very low electron phonon resistivity even at relatively low carrier concentration [26] , hence high DC conductivity is achieved with low optical conductivity below the visible range. In addition to elucidating the limits of conductivity and transparency in ultrathin graphite, we expect that the experimental techniques developed here will be broadly useful for studying the intercalation dynamics and correlated optoelectronic properties of other 2D nanomaterials that can be intercalated electrochemically. Devices for optoelectronic and transport measurements To simultaneously study the electrical and optical properties of Li-intercalated ultrathin graphite, we design a sandwich-structured cell with electrolyte (1 M LiPF 6 in w/w=1/1 ethylene carbonate/diethyl carbonate) that is sealed by bottom and top layers of thin transparent glass. Ultrathin graphite and the lithium source are deposited on the bottom glass layer and connected to separate electrical contacts. Two types of devices are fabricated for our optoelectronic ( Fig. 1a–c ) and electrical transport ( Fig. 1d–f ) measurement. Details of the device fabrication are given in the Methods section. In this planar nanoscale half-cell battery (planar nanobattery), Li metal is used as the counter electrode and ultrathin graphite as the working electrode. The intercalation process is controlled by a BioLogic SP-150 electrochemical workstation and the voltage of the planar nanobattery can be measured simultaneously during the electrochemical Li intercalation ( Supplementary Fig. 1 ). The thickness of the ultrathin graphite is determined by an atomic force microscope before cell capsulation. 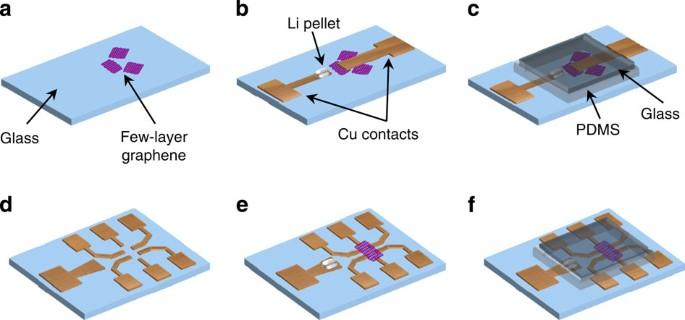Figure 1: Device schematics. (a–c) Schematic of the fabrication process of planar nanobattery devices forin situoptoelectronic measurement. (d–f) Schematic of the fabrication process of devices for electrical transport measurements. See also Methods for details of device fabrication. Figure 1: Device schematics. ( a – c ) Schematic of the fabrication process of planar nanobattery devices for in situ optoelectronic measurement. ( d – f ) Schematic of the fabrication process of devices for electrical transport measurements. See also Methods for details of device fabrication. Full size image In situ optoelectronic measurement The transmittance at a particular wavelength of pristine and Li-intercalated ultrathin graphite can be characterized by analysing the grey-scale images acquired by transmission optical microscopy (Nikon Eclipse Ti-U) using a broadband light source (Thermo Oriel), a monochromator (Spex 500 M), and a charge-coupled device (CCD) camera. A schematic of the in situ transmittance measurement system is shown in Fig. 2a (also see Methods). A series of optical images (550 nm illumination) corresponding to different intercalation stages are shown in Fig. 2d–i , along with a schematic of the lattice structure of LiC 6 ( Fig. 2h ). A clear increase in the transmittance on intercalation can be seen from Fig. 2e–g (also see Supplementary Fig. 2 and Supplementary Movie 1 ), as discussed below in detail. Furthermore, the optical transmittance change is highly reversible, as shown in Fig. 2i (also see Supplementary Fig. 3 ). 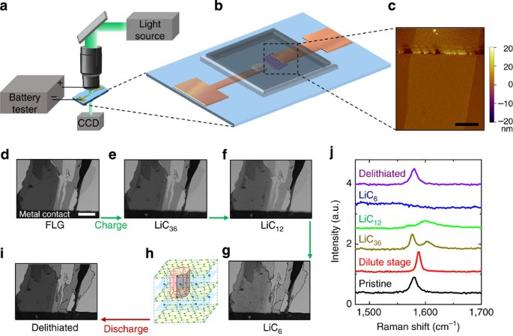Figure 2:In situoptical and electrochemical measurement with a planar nanobattery platform. (a–c) Electrochemical battery tester and transmission optical microscope are integrated (a) forin situmeasurement of individual ultrathin graphite sheets on glass substrates (b). (c) An atomic force microscope image of a uniform ultrathin graphite sheet attached to the electrical contact. Scale bar, 10 μm. (d–i) Transmission optical microscope images of ultrathin graphite before intercalation and at different intercalation stages as indicated in the figure panels. A schematic of the LiC6lattice structure is also shown in (h). The scale bar indis 100 μm. (j) Raman spectra of Li-intercalated ultrathin graphite at different intercalation stages as indicated in the figure panel. Figure 2: In situ optical and electrochemical measurement with a planar nanobattery platform. ( a – c ) Electrochemical battery tester and transmission optical microscope are integrated ( a ) for in situ measurement of individual ultrathin graphite sheets on glass substrates ( b ). ( c ) An atomic force microscope image of a uniform ultrathin graphite sheet attached to the electrical contact. Scale bar, 10 μm. ( d – i ) Transmission optical microscope images of ultrathin graphite before intercalation and at different intercalation stages as indicated in the figure panels. A schematic of the LiC 6 lattice structure is also shown in ( h ). The scale bar in d is 100 μm. ( j ) Raman spectra of Li-intercalated ultrathin graphite at different intercalation stages as indicated in the figure panel. Full size image Our transparent planar nanobattery setup also allows further characterization using Raman microscopy. As shown in Fig. 2j , we examined a series of in situ Raman spectra (Horiba Jobin Yvon with a 633 nm He-Ne laser source), which correspond to different stages of Li-graphite intercalation, with more details discussed in the Supplementary Methods II ( Supplementary Fig. 4 ). The result from our ultrathin graphite samples agrees well with previous studies of bulk samples [27] , confirming Raman microscopy as one of the tools for differentiating lithiation stages in ultrathin graphite. We also observed an in situ transmittance change of Li-intercalated ultrathin graphite at different Li x C stages by charging the Li-graphite nano-batteries ( Fig. 3a ), with a constant charging current. The black line represents a typical voltage profile of the Li-graphite nanobattery and the red, green, blue open circles depict the transmittance evolution of ultrathin graphite sheets (dotted regions in the inset of Fig. 3a ) with different thicknesses during Li-graphite intercalation. The voltage initially drops rapidly with time until it reaches 0.8 V, where an obvious slope change in the voltage profile is observed. This is due to the decomposition of the electrolyte and a solid electrolyte interphase formation [11] , [27] . No obvious change in the transmittance of the ultrathin graphite samples is observed for voltages greater than 0.2 V. A sudden increase in the transmittance (18-layer graphite from 74.4 to 77.2%, 38-layer graphite from 55.9 to 59.2%) occurs after 0.2 V, which we identify with the formation of LiC 36 (stage IV) [28] from ultrathin graphite sheets. From 0.2 to 0.1 V, a gradual change in the transmittance is observed, presumably due to the formation of LiC 27 and LiC 18 (ref. 28 ). As time increases, a second plateau appears in the voltage at ~0.1 V, which we identify with the formation of LiC 12 (stage II). At the end of the 0.1 V plateau, we expect that the entire sample has been converted to LiC 12 , and the transmittance dramatically increased to 85.8% (18-layer) and 71.9% (38-layer). A third voltage plateau appears at a value of ~0.05 V, indicating the formation of LiC 6 (stage I). At this stage, the transmittance of the 18-layer sample has increased to 90.9%, and the 38-layer sample has increased to 79.2%. Only two distinct stages are observed for the three-layer sample (from 94.5 to 95.2%, and finally 97.7%), consistent with the fact that there are only two interstitial galleries and hence only stage I and stage II are meaningfully defined. 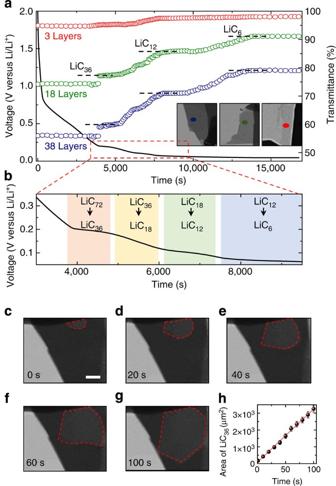Figure 3: Optical transmittance evolution during electrochemical Li intercalation process. (a) Optical transmittance (right) and electrochemical potential (left) versus lithiation time are plotted. (b) Detail of voltage profile versus time near the intercalation plateau. (c–g) Optical images of an ultrathin graphite sheet at different time points during intercalation as indicated in each panel, showing a clear lithiation front (red dashed line) between LiC36(lighter contrast) and LiC72(darker contrast). The ultrathin graphite sample is about 120 layers thick and the scale bar incis 20 μm. (h) Lithiated LiC36area versus time extracted from images such asc–g. Figure 3b shows the low potential region of the potential versus time trace in which the distinct potential plateaus can be seen more clearly. Figure 3: Optical transmittance evolution during electrochemical Li intercalation process. ( a ) Optical transmittance (right) and electrochemical potential (left) versus lithiation time are plotted. ( b ) Detail of voltage profile versus time near the intercalation plateau. ( c – g ) Optical images of an ultrathin graphite sheet at different time points during intercalation as indicated in each panel, showing a clear lithiation front (red dashed line) between LiC 36 (lighter contrast) and LiC 72 (darker contrast). The ultrathin graphite sample is about 120 layers thick and the scale bar in c is 20 μm. ( h ) Lithiated LiC 36 area versus time extracted from images such as c – g . Full size image The changes in optical transmission in our planar nanobattery allow a direct observation of the lithiation process on an individual ultrathin graphite sheet with excellent spatial and temporal resolution. As shown in Fig. 3c–g , a clear lithiated (LiC 36 ) and dilute stage (LiC 72 ) interface (that is, a lithiation front) is observed within 100 s, and the lithiated area becomes more transparent and the LiC 36 area increases linearly with time ( Fig. 3h ). This agrees well with our electrochemical testing scheme with a constant current charge/discharge process. Thus, our integrated system provides a powerful tool to investigate the intrinsic lithiation kinetics in the two-phase reaction at the nanoscale [29] . Thickness and wavelength dependence We next consider the layer number and wavelength dependence of the in situ optical transmission of individual ultrathin graphite sheets. In Fig. 4a–c , the wavelength dependence of the transmittance is shown in the visible range from 400 to 800 nm for samples of various thicknesses. For pristine ultrathin graphite ( Fig. 4a ), the transmittance is weakly dependent on the wavelength, consistent with previous reports [6] ; the absorption by ultrathin graphite is approximately Nπα ( πα =2.3%), where α is the fine structure constant and N the number of graphene layers. This absorption results from interband transitions in the Dirac spectrum of graphene, which give a nearly constant optical conductivity σ ≈ πe 2 /2 h where e is the elemental charge and h Planck’s constant. For LiC 12 stage ( Fig. 4b ), the transmittance depends more strongly on wavelength, increasing the most for longest wavelengths. For the LiC 6 stage ( Fig. 4c ), the wavelength-dependent transmittance shows a maximum around 500 nm, and the transmittance of LiC 6 is still higher compared with pristine ultrathin graphite. Interestingly, the transmittance of LiC 6 still increases compared with LiC 12 for wavelengths well below the maximum, while above the transmittance maximum the LiC 6 transmittance decreases compared with LiC 12 . 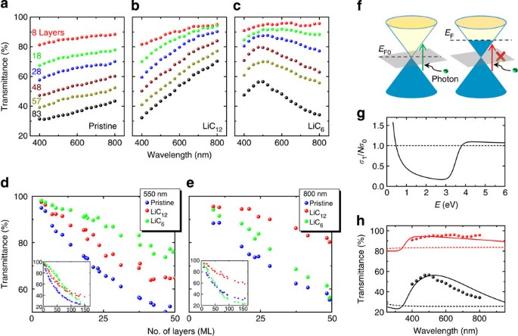Figure 4: Wavelength-dependent optical transmittance of intercalated ultrathin graphite. (a–c) Transmittance as a function of wavelength for different thickness ultrathin graphite samples for pristine ultrathin graphite (a), LiC12(b), LiC6(c) stages. (d–e) Transmittance as a function of thickness for pristine ultrathin graphite, LiC12, and LiC6at wavelengths 550 nm (d) and 800 nm (e). Insets show transmittance at same wavelength over a larger range of thicknesses. (f) Schematic of doped graphene band structure illustrating suppression of optical transitions due to Pauli exclusion principle. (g,h) Modelled results for the real part of optical conductivity,σ1/Nσ0(g), and transmittance (h) of pristine ultrathin graphite (dashed line) and intercalated LiC6(solid line). For the model, we assumeEF=1.5 eV,n=1.5,T=300 K and 1/τ=γ=200 cm−1. The red and black colours in (h) correspond to 8 and 83-layer ultrathin graphite sheets, respectively. Experimental data for 8 and 83-layer graphite shown incare also plotted inhfor comparison with the model. Figure 4: Wavelength-dependent optical transmittance of intercalated ultrathin graphite. ( a – c ) Transmittance as a function of wavelength for different thickness ultrathin graphite samples for pristine ultrathin graphite ( a ), LiC 12 ( b ), LiC 6 ( c ) stages. ( d – e ) Transmittance as a function of thickness for pristine ultrathin graphite, LiC 12 , and LiC 6 at wavelengths 550 nm ( d ) and 800 nm ( e ). Insets show transmittance at same wavelength over a larger range of thicknesses. ( f ) Schematic of doped graphene band structure illustrating suppression of optical transitions due to Pauli exclusion principle. ( g , h ) Modelled results for the real part of optical conductivity, σ 1 / Nσ 0 ( g ), and transmittance ( h ) of pristine ultrathin graphite (dashed line) and intercalated LiC 6 (solid line). For the model, we assume E F =1.5 eV, n =1.5, T =300 K and 1/ τ = γ =200 cm −1 . The red and black colours in ( h ) correspond to 8 and 83-layer ultrathin graphite sheets, respectively. Experimental data for 8 and 83-layer graphite shown in c are also plotted in h for comparison with the model. Full size image Figures 4d,e show the optical transmittance for pristine and intercalated ultrathin graphite sheets as a function of layer number. For both 550 and 800 nm, a clear increase of the optical transmittance is seen after intercalation, both for LiC 12 and LiC 6 . For 550 nm wavelength ( Fig. 4d ), the transmittance increases monotonically with Li concentration; for LiC 6 versus pristine ultrathin graphite, the transmittance increase can be as high as 55% (for a sample of 60–80 layers). For 800 nm wavelength ( Fig. 4e ), the transmittance for all measured thicknesses first increases (LiC 12 ) and then decreases (LiC 6 ); for LiC 12 versus pristine ultrathin graphite, the transmittance has an increase up to twofold (for a sample more than 100 layers). We also observed that in thicker sheets (insets of Fig. 4d,e ), the transmittance of LiC 6 increases less and starts to approach the value of its pristine state at both wavelengths of 550 and 800 nm, that is, at 550 nm for 90-layer thickness the transmittance at LiC 6 state starts to approach the value of LiC 12 state and approaches the value of pristine state at about 150 layers, and for 800 nm wavelength the transmittance of LiC 6 becomes lower than the value of pristine state with layer number greater than 60. In situ optical measurements in reflective mode are also shown in Supplementary Fig. 5 , further confirming the wavelength-dependent optical properties of lithiated ultrathin graphite. Drude and interband contribution The changes in optical transmittance in the visible range described above can be qualitatively understood as follows. The result of the Li intercalation is electron doping due to the low electrochemical potential of Li metal. As shown in Fig. 4f , intercalation of Li heavily dopes the ultrathin graphite, shifting up the Fermi level. The magnitude of Fermi level shift is associated with the carrier density, which increases monotonically with lithium concentration. The doping concentration is as high as ~6 × 10 14 cm −2 per layer for LiC 6 , corresponding to E F ≈1.5 eV [30] , higher than the highest doping that can be achieved in graphene with electrolytic gating [24] . The increase in Fermi energy leads to the suppression of interband optical transitions for photon energies ω <2 E F , thus decreasing the optical conductivity and increasing the transmission. As doping increases, however, intraband (Drude) conductivity becomes important, decreasing the transmission for ħω<ħ/τ (where τ is the carrier relaxation time) due to the electron–longitudinal optical (LO) phonon interaction. Thus, we expect that the transmission of ultrathin graphite is enhanced with doping for a window of photon energies ħ/τ<ħω <2 E F . This phenomenon has been observed previously in gated monolayer and FLG samples, where doping levels were much lower than explored here and the window occurred in the infrared [31] . A decrease in the absorption coefficient is also observed in graphite intercalation compounds by Hennig et al. [19] In Li-intercalated graphite, the window manifests as a minimum in reflectivity occurring near 740 nm for bulk LiC 12 and 440 nm for bulk LiC 6 (ref. 32 ). The reflectivity minimum previously observed for bulk LiC 6 corresponds reasonably well to our observation of a transmission maximum near 500 nm ( Fig. 4c ). For LiC 12 , the transmission maximum may occur at a longer wavelength than our experiment accesses, and we observe only an enhancement of long-wavelength transmission. Thus, we conclude that the overall reduction in interband transitions by Pauli blocking is responsible for the transmission increase, and the higher Drude conductivity of more strongly doped LiC 6 is responsible for the observed reduction in transmission at long wavelength and the non-monotonic doping dependence of transmission at these wavelengths. Further insight into these results is gained by examining the optical transmittance in terms of the optical conductivity. On a substrate with refractive index n , the transmittance of ultrathin graphite with optical (sheet) conductivity σ opt = σ 1 + iσ 2 , relative to that of the bare substrate, can be expressed as [33] : where Z 0 is the free space impedance. Li et al. [31] and Stauber et al. [34] reported the optical conductivities of doped monolayer graphene in the IR range. For ħω <2 E F , that is, below the Pauli blocking edge, σ 1 >> σ 2 ; σ 1 is large due to LO phonon emission and σ 2 passes through zero near the plasma edge ( ε 1 =0; also see the Supplementary Methods IV ) so that the transmission reaches a maximum. Therefore, near the transmission maximum, σ opt ~ σ 1 . We then modelled the optical transmittance based on optical conductivity with a Drude contribution from the free carriers and an interband contribution that turns on for ħ ω>2 E F due to Pauli unblocking, that is, σ opt (ω)= σ D + σ ib . The conductivity is modelled as N layers of graphene. The Drude sheet conductivity can be written as [2] , where n 2D is the carrier density per layer, m the effective mass, γ =1/ τ is the carrier relaxation rate, and N is the number of layers. The thermal broadening of the Pauli blocking leads to [35] , and the imaginary part of σ ib is obtained from Kramers–Kronig relation. The details of the modelling are presented in the Supplementary Methods IV . Figure 4g shows a schematic of σ 1 / Nσ 0 versus the photon energy from the model for N -layer ultrathin graphite before and after Li intercalation. σ 1 in the visible range significantly decreases on Li intercalation, which leads to a large increase in the optical transmittance. The modelled transmittances of both 8-layer and 83-layer ultrathin graphite ( Fig. 4h , solid curves) closely resemble the corresponding experimental data, and the sharpening of the transmission maximum for thicker films is a consequence of the plasma edge as discussed in the Supplementary Methods IV ( Supplementary Fig. 6 ). Electrical properties In order to understand the prospects for highly transparent Li-intercalated ultrathin graphite for conducting transparent electrode applications, we adapted our planar nanobattery setup for in situ conductivity measurements of ultrathin graphite during electrochemical cycling. We transferred ultrathin graphite onto predeposited electrical contacts in a Hall-bar arrangement ( Fig. 5a inset, see also Supplementary Figs 7–9 ). 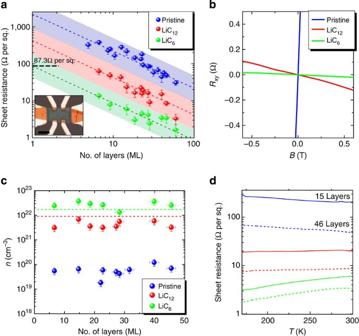Figure 5: Transport measurement of Li-intercalated ultrathin graphite sheets. (a) Resistivity versus thickness for ultrathin graphite sheets with different thickness. Data for pristine (red) and two lithiated stages (LiC12and LiC6indicated as green and blue) are shown. Inset: an optical image of an ultrathin graphite device with Hall-bar geometry before intercalation. The scale bar is 10 μm. (b) Hall resistance of a 4-nm-thick pristine FLG sheet and its LiC12and LiC6states as a function of magnetic field. (c) Carrier density calculated from Hall measurement as a function of ultrathin graphite thickness. (d) Temperature-dependent sheet resistance for two ultrathin graphite samples. Blue, red and green colours indicate pristine, LiC12and LiC6stages, respectively. Figure 5a shows the room temperature sheet resistance R s for ultrathin graphite samples with different thickness before intercalation as well as intercalated to LiC 12 and LiC 6 . As expected, all intercalated ultrathin graphite samples invariably exhibit a lower resistivity compared with their pristine state (also see Supplementary Fig. 10 ). Note that R S measured on both stage I and II is inversely proportional to the sample thickness (before intercalation) as indicated by the dashed lines. Considering the expansion of the graphite-layer spacing during Li intercalation [36] , we can estimate that ρ (LiC 6 )~3.1 × 10 −6 and ρ (LiC 12 )~1.4 × 10 −5 Ω cm −1 . The intrinsic limit of the conductivity for doped graphene at room temperature is set by electron–acoustic phonon scattering and is approximately σ dc,phonon =33 mS per layer [26] , [37] for Fermi energies in the linear portion of the band structure, while we observe a DC sheet conductivity σ dc ≈11 mS per layer in LiC 6 . At the high doping levels present in LiC 6 , we expect significant band curvature and reduction in the Fermi velocity, likely reducing the limiting conductivity. In addition, disorder may play a role. Thus, our approach within a factor of ~3 to the limiting conductivity value for the graphene Dirac band is impressive. Figure 5: Transport measurement of Li-intercalated ultrathin graphite sheets. ( a ) Resistivity versus thickness for ultrathin graphite sheets with different thickness. Data for pristine (red) and two lithiated stages (LiC 12 and LiC 6 indicated as green and blue) are shown. Inset: an optical image of an ultrathin graphite device with Hall-bar geometry before intercalation. The scale bar is 10 μm. ( b ) Hall resistance of a 4-nm-thick pristine FLG sheet and its LiC 12 and LiC 6 states as a function of magnetic field. ( c ) Carrier density calculated from Hall measurement as a function of ultrathin graphite thickness. ( d ) Temperature-dependent sheet resistance for two ultrathin graphite samples. Blue, red and green colours indicate pristine, LiC 12 and LiC 6 stages, respectively. Full size image In order to elucidate the type and density of charge carriers, we investigated the Hall resistance at perpendicular magnetic fields. The linear R xy ( B ) curves with negative slope ( Fig. 5b ) indicate that charge carriers are electrons for a 4-nm thick FLG device after Li intercalation. The carrier density n H is readily determined by a measurement of the Hall coefficient R H = R xy /B , where R H is related to n H by n H =1/e R H . With the information of expanded thickness of Li-intercalated ultrathin graphite, our measurements reveal that bulk n H ranges from 3 × 10 21 to 7 × 10 21 cm −3 for LiC 12 and from 1.5 × 10 22 to 3.5 × 10 22 cm −3 for LiC 6 , with no observable dependence on sample thickness, as shown in Fig. 5c . These values compare reasonably well with the full ionization values of 1.7 × 10 22 cm −3 for LiC 6 and 9.0 × 10 21 cm −3 for LiC 12 , which are indicated in Fig. 5c as guidelines. Figure 5d shows the temperature dependence of the sheet resistance. R s ( T ) is metallic, that is, R S decreases with decreasing T, for samples at LiC 6 state, while LiC 12 exhibits a moderate temperature dependence, and pristine samples always exhibited weakly non-metallic behaviour consistent with previous studies [3] . The strong decrease in R S with lowering T for LiC 6 is consistent with phonon-limited conduction and further corroborates that we have approached the phonon-limited conductivity in Li-intercalated ultrathin graphite [21] . Transparent electrode performance In the race to find better transparent electrodes, researchers have investigated numerous candidate materials [25] , [38] , [39] , [40] , [41] . 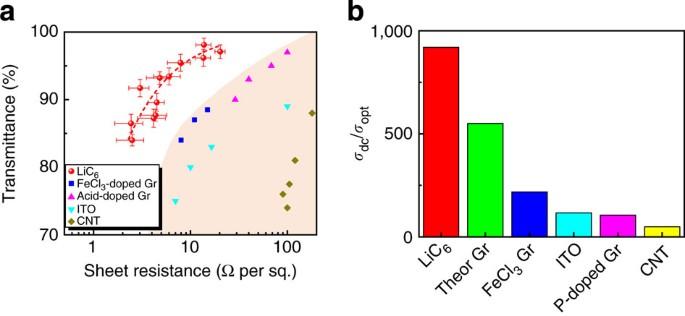Figure 6: Optoelectronic properties of intercalated ultrathin graphite sheets and comparison with other materials. (a) Transmittance at 550 nm versus sheet resistance for our LiC6FLG, and other high-performance carbon-based transparent conducting materials FeCl3-doped graphene15, acid-doped graphene9and carbon nanotube (CNT) films38, as well as indium tin oxide (ITO)40. The red solid line is a fit with equation 3 withσdc/σopt=920±100. (b) FOM (σdc/σopt) for various materials. A higher value forσdc/σoptleads to a better performance in transparent conductor. Figure 6a shows the transmittance versus sheet resistance of Li-intercalated ultrathin graphite as well as other high-performance transparent conducting materials, including other carbon-based materials [15] , [42] , and the best commercial indium tin oxide electrodes [40] , [43] . In previous doped graphene studies, an improvement in the electrical conductivity was observed; however, little or no change of transmittance in the visible range was obtained [9] , [15] . When σ 1 >> σ 2 and n =1, to compare the performance of a freestanding film in vacuum, Equation (1) becomes: Figure 6: Optoelectronic properties of intercalated ultrathin graphite sheets and comparison with other materials. ( a ) Transmittance at 550 nm versus sheet resistance for our LiC 6 FLG, and other high-performance carbon-based transparent conducting materials FeCl 3 -doped graphene [15] , acid-doped graphene [9] and carbon nanotube (CNT) films [38] , as well as indium tin oxide (ITO) [40] . The red solid line is a fit with equation 3 with σ dc / σ opt =920±100. ( b ) FOM ( σ dc / σ opt ) for various materials. A higher value for σ dc / σ opt leads to a better performance in transparent conductor. Full size image where the sheet resistance is R s =1/ σ dc . Thus, at a given sheet resistance, the transmission is determined by the ratio σ dc / σ opt , which can be used as the Figure of Merit (FOM) to characterize the performance of a transparent conductor. As shown in Fig. 6a , we fit the data for our Li-intercalated FLG devices to Equation (1) using σ dc / σ opt as a fitting parameter, and fitting result gives σ dc / σ opt =920 (fitting details also see Supplementary Figs 11 and 12 ). For the best sample at LiC 6 state, we measured transmittance of 91.7% and 3.0 Ω per sq, obtaining σ dc / σ opt =1400. Figure 6b shows the best measured σ dc / σ opt for the material systems shown in Fig. 6a ; σ dc / σ opt for our LiC 6 exceeds that of FeCl 3 -intercalated FLG ( σ dc / σ opt =235) [15] and the best commercial transparent electrode indium tin oxide ( σ dc / σ opt =118) [40] . In fact, σ dc / σ opt of few-layer LiC 6 exceeds that for all other carbon-based materials, and as far as we can determine, it is the highest for any uniform thin film. Higher transparency at a given conductivity has only been achieved in inhomogenous conductors such as metal nanowire networks [44] , which may not be suitable for many applications. It also exceeds the intrinsic limit for doped graphene [9] , [25] , [38] previously expected ignoring the increased transparency due to Pauli blocking. The sheet resistance and transparency easily meet the need for optoelectronic device applications where 90% and 10 Ω per sq is required. Thus, we expect that electrochemically intercalated FLG is promising for applications where the highest DC conductivity at a given optical transparency is needed. To demonstrate the feasibility of ultrathin graphite as transparent electrode for industrial applications, we successfully fabricated stable millimeter-scale devices using encapsulated commercially obtained CVD-grown thin graphite (see Methods and Supplementary Fig. 13 ). Comparison of two 40- and 80-nm thick devices before and after Li intercalation are shown in Fig. 7a,b . Transmittance spectra are also characterized before and after Li intercalation, as shown in Fig. 7c , which are very similar to the results of single exfoliated ultrathin graphite sheets. Changes in the sheet resistance was also measured for 40-nm-thick devices by the Van der Pauw method (see Supplementary Fig. 14 ). The sheet resistances of three different devices dropped drastically on complete lithiation from 35.4, 47.7, 57.0 Ω per sq (graphite) to 3.0, 3.9, 1.7 Ω per sq (LiC 6 ), respectively. The 1.7 Ω per sq correspond to a single layer sheet resistance of 200 Ω per sq, only 2.3 times larger than the single flake value (87.3 Ω per sq) from our experiment, leads to a FOM of 400. 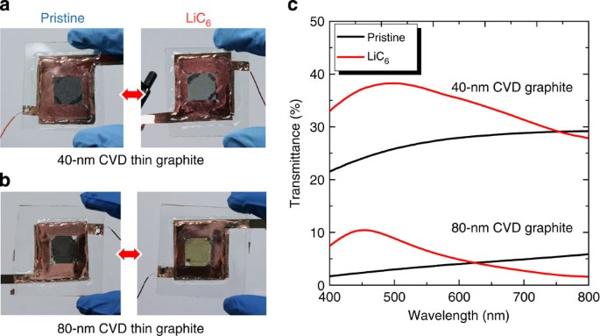Figure 7: Demonstration of encapsulated large-area transparent electrode (a,b) Photographs of 40- and 80-nm thick CVD-grown thin graphite before and after full Li intercalation. (c) Corresponding transmittance spectra of the two devices before and after full intercalation. Figure 7: Demonstration of encapsulated large-area transparent electrode ( a , b ) Photographs of 40- and 80-nm thick CVD-grown thin graphite before and after full Li intercalation. ( c ) Corresponding transmittance spectra of the two devices before and after full intercalation. Full size image We discuss the ultimate limits to conductivity and transparency of doped graphene-based systems. Previous studies [25] of graphene as a transparent conductor have ignored changes in the optical conductivity, assuming it remains limited by interband transitions and is fixed at σ opt = σ ib ≈ N π e 2 /2 h=Nσ 0 , with N the number of layers, as discussed above. For phonon-limited conduction at room temperature, σ dc = Nσ dc,phonon where. σ dc,phonon =33 mS [26] , [37] . This predicts a maximum value of σ dc / σ opt ≈550, while our intercalated ultrathin graphite significantly exceeds this value. However, as noted previously, below the Pauli blocking edge σ opt is the free carrier Drude conductivity that can be smaller than σ ib . Optical measurements on doped monolayer graphene gives f ≡ σ 1 / σ 0 ≈0.3 below the interband edge for E F ≈0.3 eV [31] . Assuming this value of f implies σ dc / σ opt ≈1,800 in reasonable agreement with our best observation; however, there are no experimental results on the magnitude of σ 1 and hence f for the E F ≈1.5 eV conditions of our intercalated graphene. Theory predicts that the Drude optical conductivity for frequencies above the LO phonon frequency is limited by the electron–LO phonon relaxation rate, γ =1/ τ LO (ref. 34 ). At the higher E F of our experiments, the electron phonon scattering rate will be stronger because of the larger electronic density of states (~ E F ), but the high frequency Drude conductivity falls off as σ 1 ~ E F γ /( γ 2 + ω 2 )~ E F γ / ω 2 . This suggests that σ 1 and hence f at ω ≤2 E F are approximately independent of E F so that f ≡ σ 1 / σ 0 ≈0.3 may also be valid at E F ≈1.5 eV, and our estimate of the intrinsic limit of σ dc / σ opt ≈1,800 is reasonable. Thus, we believe that our real devices approach the ultimate limits of transparency at a given conductivity for the doped graphene system. In summary, we have designed a methodology via a planar nanobattery for in situ study of the electrical and optical properties of individual ultrathin graphite sheets during electrochemical intercalation and deintercalation. Metallic-like temperature-dependent transport is observed in Li-intercalated ultrathin graphite with conductivities approaching the acoustic phonon limit at room temperature and is comparable to good metals. Due to the unusual band structure of graphene, Li intercalation can simultaneously increase the DC electrical conductivity and increase optical transmission in the visible, allowing Li-intercalated FLG to achieve an unprecedented FOM σ dc / σ opt =920, significantly higher than any other material and approaching the ultimate limit expected for doped graphene systems. Our technique will allow similar studies to be carried out in other 2D materials. Furthermore, the methodology reported in this study can be applied to in situ investigations of the intercalation process with good spatial and temporal resolution in materials for electrochemical energy storage applications. Device fabrication for electrochemical/optical measurements Pristine ultrathin graphite sheets from monolayer to 50 nm (~150 layers) are first obtained by mechanical exfoliation of Kish graphite onto 0.2 mm thick glass substrates (Fisher Scientific), followed by deposition of electrical contacts (50 nm copper) on top of the selected ultrathin graphite sheets using a shadow mask technique in electron beam evaporator. The device is then transferred into a glove box filled with argon gas, and a small lithium pellet is deposited onto an isolated electrical contact, followed by the addition of a small amount of electrolyte (LiPF 6 in EC:DEC w-w=1:1) to cover the region with both ultrathin graphite and lithium pellet. At last, the centre region with electrolyte/lithium/ultrathin graphite is covered by another piece of 0.2 mm thick glass and sealed by polydimethylsiloxane, as shown in Fig. 1c . Device fabrication for electrical transport measurements During the Li intercalation process, the volume of ultrathin graphite gradually expands because of the insertion of lithium atoms. The layer spacing of LiC 6 is ~10% larger than that of pristine graphite [36] . Therefore, the narrow metal electrodes fabricated by the normal method of thermal evaporation on top of ultrathin graphite usually crack after intercalation. Here, we use a lithography-free fabrication method shown in Fig. 1d–f . The 50-nm thick copper Hall-bar/lithium-contact electrodes are prepatterned on a blank glass wafer. A uniform exfoliated ultrathin graphite sheet is then transferred onto the top of the electrodes aligned by a micromanipulator. The rest of the device fabrication is the same as described above. Using this method, ultrathin graphite sheets are attached to the top of the electrodes and can expand freely during Li intercalation. Fabrication of large-scale CVD graphene devices CVD ultrathin graphite on nickel foil (2″ × 2″) is obtained from Graphene Supermarket and cut into 1.5 × 1.5 cm pieces. A solution based (1 M FeCl 3 in deionized water as etchant, Sigma Aldrich) etching/transfer method is then carried out to transfer ultrathin graphite onto transparent substrates (for example, glass and polyethylene terephthalate). A gel electrolyte film is prepared by mixing P (VDF-HFP)/Acetone/deionized water (w:w:w=1:19:1, Sigma Aldrich) as a mixed solution. The electrolyte is then drop-cast on glass and ready for use after drying in a vacuum oven (MTI Corp.). A sandwiched device structure of glass/ultrathin graphite/gel electrolyte/polyethylene terephthalate is assembled in an argon-filled glove box. The transmittance of the device is measured by a UV–vis spectrometer (PerkinElmer Lambda 35). In situ optical transmission measurements A system based on a transmission optical microscope (Nikon Eclipse Ti-U) combined with a CCD camera is used to acquire transmission data. Microscope objectives with × 5 and × 20 magnification are used depending on the size of the sample. A beam of light at particular wavelength from a monochromator (Spex 500 M, 0.2 nm bandwidth) passes through the transmission optical microscope and is then projected onto the 1,392 × 1,040 lines of the grey CCD camera. Intensity is then extracted from images taken by CCD camera and is normalized to the signal obtained through a region of bare substrate close to the sample to give the transmission at that wavelength. Such analysis results in a weak overestimate of transmittance for ultrathin graphite embedded in an electrolyte solution; however, if we focus on the highly transparent samples (more than 90%), the difference is negligible (~1%). Electrochemical control An electrochemical workstation (Biologic SP-150) is used to control charge/discharge of the Li-ultrathin graphite nanobattery and measure the time-dependent potential on intercalation (lithiation) and deintercalation (delithiation). Details are also discussed in Supplementary Methods I . How to cite this article: Bao, W. et al. Approaching the limits of transparency and conductivity in graphitic materials through lithium intercalation. Nat. Commun. 5:4224 doi: 10.1038/ncomms5224 (2014).